Polariton-generated intensity squeezing in semiconductor micropillars The generation of squeezed and entangled light fields is a crucial ingredient for the implementation of quantum information protocols. In this context, semiconductor materials offer a strong potential for the implementation of on-chip devices operating at the quantum level. Here we demonstrate a novel source of continuous variable squeezed light in pillar-shaped semiconductor microcavities in the strong coupling regime. Degenerate polariton four-wave mixing is obtained by exciting the pillar at normal incidence. We observe a bistable behaviour and we demonstrate the generation of squeezing near the turning point of the bistability curve. The confined pillar geometry allows for a larger amount of squeezing than planar microcavities due to the discrete energy levels protected from excess noise. By analysing the noise of the emitted light, we obtain a measured intensity squeezing of 20.3%, inferred to be 35.8% after corrections. While very efficient sources of non-classical light, essentially based on bulk nonlinear crystals, have been developed in the last 20 years, the quest for integrated quantum sources is a major challenge for the cutting edge research activity in the field of quantum information technologies. Successful examples in the discrete variable regime are represented by efficient single and entangled photons sources in semiconductor quantum dots [2] , [3] , [4] . Photon antibunching and squeezing were theoretically predicted and experimentally demonstrated in pioneering resonance fluorescence experiments [5] , [6] , [7] , [8] . In strong contrast, despite several theoretical proposals [9] , [10] , the continuous variables regime has seen so far only very few experimental achievements [11] , [12] , [13] of squeezed states of light in semiconductor materials. Here, for the first time in this type of systems, we achieve a high degree of intensity squeezing exploiting an effective Kerr effect for microcavity polaritons. Let us note that, due to the giant polariton nonlinearities [14] , the power range used here (5–20 mW) is two orders of magnitudes lower than in previous experiments [11] . These results open the way to the implementation of ultra-low threshold quantum devices integrated in a semiconductor platform. Exciton-polaritons are half-light half-matter bosonic particles arising from the strong coupling between excitons and photons in semiconductor microcavities [15] . They exhibit strong nonlinearities due to the Coulomb interactions of their excitonic part, responsible for the rich variety of quantum effects recently unveiled [16] , ranging from Bose–Einstein condensation [17] and superfluidity [18] , [19] to more complex phenomena such as dark and bright solitons [20] , [21] , magnetic monopole-like half-solitons [22] , half-vortices [23] and vortex lattices [24] . The great potential of polaritons for non-classical fields generation was recognized very soon after the experimental demonstration of the coherent nonlinear optical response of microcavity polaritons allowing for the observation of parametric amplification and oscillation in such systems [25] , [26] , [27] . Especially interesting is the case of degenerate polariton four-wave mixing in which the strong nonlinearities originating in the polariton–polariton interactions allow describing the polariton system as an effective Kerr medium whose refractive index depends on the light intensity [13] , [28] , [29] . Kerr media are well known to be very efficient sources of quadrature-squeezed light. Indeed, quadrature squeezing of about 4% was observed in a planar semiconductor microcavity, by using degenerate polariton four-wave mixing in 2004 (ref. 11 ). Despite several attempts with specifically designed planar microcavity samples, significant improvements of this first result were prevented by the excess noise coming from the intrinsic multimode nature of the emission in a planar microcavity, which is characterized by a continuum of polariton modes and is favourable to the coupling with lattice phonons. Very recently, it has been predicted [30] that a large amount of squeezing could be achieved by quantizing the in-plane polariton field modes via a geometric confinement (strong localization limit [30] ). This tight confinement separates the modes energetically, severely reducing any nonlinear multimode coupling responsible for increased excess noise and reduced quantum effects. In this paper, we apply this method in a controlled way making use of semiconductor micropillars [31] , [32] and we demonstrate up to 20.3% of directly measured squeezing in the amplitude quadrature of the emitted light. Experimental configuration In our set-up, the pillars are fabricated by etching a λ GaAs microcavity containing two GaAs–InGaAs quantum wells, resulting in a polariton Rabi splitting of about 4 meV. The cavity finesse is of the order of 700, which gives a 0.1 meV polariton linewidth. 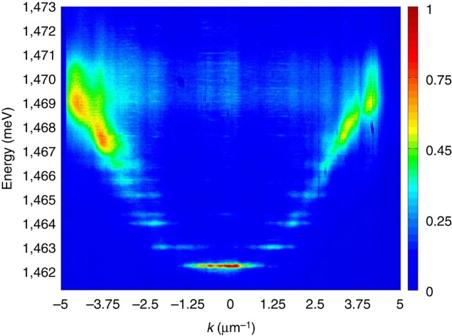Figure 1: Energy modes separation. Dispersion curve for the 6 μm circular pillar used in the experiment (−5 meV cavity detuning), obtained with a non-resonant pumping at 1, 550 meV. The lower polariton branch with several spatial modes and the weakly excited upper branch are visible. The modes are energetically separated and squeezing is protected against multimode nonlinear coupling. Figure 1 shows the energy separation of the polariton modes due to the finite size of the pillar. As shown in Fig. 2a the cavity mirrors are asymmetric with the bottom Bragg mirror twice thicker than the top one (30 pairs of Al 0.1 Ga 0.9 As−Al 0.95 Ga 0.05 As versus 15 pairs for the top mirror), optimizing the cavity for experiments in reflection configuration. The cavity is wedged in one direction, providing a large choice of cavity–exciton detuning by selecting pillars placed in different positions on the chip. We can choose the shape and size of the micropillars in order to engineer the spatial distribution of the confined modes and their energy separation. 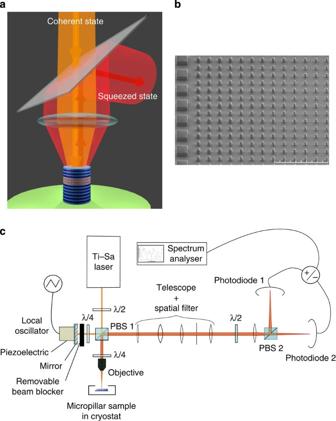Figure 2: Sample and set-up. (a) Principle of squeezed light production with a pillar-shaped microcavity. The microcavity is made of a pair of quantum wells (white-red-white layers) sandwiched by two Bragg mirrors (alternation of light blue and dark blue layers); the green layer is the substrate. The orange beam represents the pump laser arriving on the sample at normal incidence, slightly blueshifted with respect to the energy of the lower polariton branch. The red beam represents the squeezed light emitted by the squeezed polariton field present in the microcavity. (b) Image of the sample obtained with scanning electron microscopy. The different shapes and sizes of the pillars are visible. The scale bar corresponds to 100 μm. (c) Scheme of the experimental set-up for the noise detection. The higher squeezing values were measured with the balanced detection set-up, realized by blocking the local oscillator with the beam blocker. The choice of adding (+) or subtracting (−) the photodiodes signals determines the measurement: intensity noise (+) or shot noise (−). To measure the noise quadratures of the field one unblocks the local oscillator and set the mixer to (−); in this case, the shot noise is measured by blocking the light reflected from the microcavity. PBS: polarizing beam splitter;,: half-wave, quarter-wave plate. Figure 2b shows the large square-shaped pillars (width of 20 μm) and small square or round-shaped pillars (width from 6 μm to 2 μm) available on the studied sample. Figure 1: Energy modes separation. Dispersion curve for the 6 μm circular pillar used in the experiment (−5 meV cavity detuning), obtained with a non-resonant pumping at 1, 550 meV. The lower polariton branch with several spatial modes and the weakly excited upper branch are visible. The modes are energetically separated and squeezing is protected against multimode nonlinear coupling. Full size image Figure 2: Sample and set-up. ( a ) Principle of squeezed light production with a pillar-shaped microcavity. The microcavity is made of a pair of quantum wells (white-red-white layers) sandwiched by two Bragg mirrors (alternation of light blue and dark blue layers); the green layer is the substrate. The orange beam represents the pump laser arriving on the sample at normal incidence, slightly blueshifted with respect to the energy of the lower polariton branch. The red beam represents the squeezed light emitted by the squeezed polariton field present in the microcavity. ( b ) Image of the sample obtained with scanning electron microscopy. The different shapes and sizes of the pillars are visible. The scale bar corresponds to 100 μm. ( c ) Scheme of the experimental set-up for the noise detection. The higher squeezing values were measured with the balanced detection set-up, realized by blocking the local oscillator with the beam blocker. The choice of adding (+) or subtracting (−) the photodiodes signals determines the measurement: intensity noise (+) or shot noise (−). To measure the noise quadratures of the field one unblocks the local oscillator and set the mixer to (−); in this case, the shot noise is measured by blocking the light reflected from the microcavity. PBS: polarizing beam splitter; , : half-wave, quarter-wave plate. Full size image The pillars are cooled down to 5 K in a cryostat mounted in reflection configuration and excited with a CW single-mode Ti:Sa laser tuned to be quasi-resonant with the ground-state level of the lower polariton branch. The laser is frequency locked to a Fabry–Perot cavity and its intensity is stabilized by means of an electro-optical modulator. The laser was verified to be at the shot noise for frequencies above 1 MHz. The spatial mode is filtered by a five meters long single-mode optical fibre shielded against thermal fluctuations. The laser beam is focused by a microscope objective treated with a near-infrared optimized coating and excites the sample at normal incidence. Upstream of the microscope objective, a motorized plate coupled with a polarizing beam splitter (PBS) allows us to finely control the pump power on the sample and a plate placed between the beam splitter and the objective ensures that the light coming on the sample is circularly polarized. With the polarized beam splitter, the plate forms an optical circulator since the light re-emitted from the sample was measured to be 95% circularly polarized, as expected from spin conservation. The light reflected from the cavity is thus collected and sent to the detectors. The shape of the laser spot on the sample is Gaussian with a waist of 5.5 μm, well matched to the round pillars with a diameter of 6 μm. In the studies presented here, we hence use a round micropillar of 6 μm, which ensures an optimal mode matching between its polaritonic ground state and the focalized excitation laser. The re-emitted light is collected by the same microscope objective and sent through a telescope and a spatial filter, allowing us to select only the light coming out of the pillar or some specific region if needed. As shown in Fig. 2c , the sample emission is collected in a set-up allowing performing both balanced and homodyne detections. For the balanced detection, the collected light is equally split into two parts by a plate associated to a a polarizing beam splitter (PBS 2) and each beam is collected by a photodiode. The high frequency (HF) outputs of the two identical photodiodes (81% quantum efficiency, with home-made low-noise electronics) are added or subtracted with a passive circuit, amplified by a low-noise, HF amplifier and sent to a spectrum analyser giving us the spectral noise power (thereafter simply called ‘noise’). The choice of addition or subtraction allows us to quickly switch between the measurement of the intensity noise (addition mode) or the shot noise (difference mode). The common mode rejection of the balanced diodes was 45 dB at 7 MHz. For the homodyne detection, a portion of the pump laser is mixed on PBS 1 with the light emitted by the micropillar with an orthogonal polarization, and acts as local oscillator. In this case, the HF output of the photodiodes are subtracted and the measured quantity gives the noise in the quadrature of the reflected field that is in phase with the local oscillator. The relative phase between the local oscillator and the reflected field is controlled with a piezoelectric-mounted mirror, allowing measuring all quadratures. The shot noise is measured by blocking the light reflected from the microcavity. For the homodyne set-up, it is important to note that the spatial mode of the sample emission can be strongly distorted by the nonlinear interactions and it is no longer Gaussian-shaped at high polariton densities. For this reason, it was found very difficult to achieve the mode matching with the local oscillator necessary to have efficient homodyne detection, except in the special case of very low detuning of the pump laser with respect to the ground-state level of the lower polariton branch (since in this case we have a low density of polariton even above threshold). There, proper homodyne detection was achieved (mode matching of 90%). However, such a low detuning is not optimal and thus the squeezing measured with the homodyne detection is lower than at the optimum detuning. Intensity squeezing measurements at the optimum pump–polariton detuning were performed with the balanced set-up. 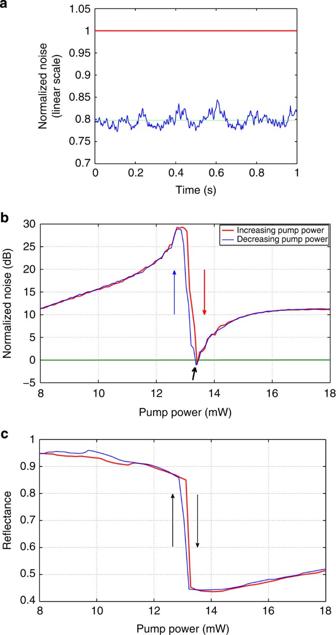Figure 3: Intensity squeezing and bistability. (a) Squeezed intensity noise at fixed pump power near the lower turning point (linear scale), on a 6 μm pillar at cavity–exciton detuning of −5 meV and a polariton–laser detuning of 0.19 meV. The noise data were normalized with a measurement of the shot noise and a measurement of the dark noise, withS(t) = (noise(t) −<dark(t)>)/(< shotnoise(t)>−<dark(t)>), <...> being the time average. The measured noise reduction is 20.3±1.5% (−1 dB) below the shot noise limit before corrections, 35.8±2.6% after. The dashed green line is the average noise and the red line is the shot noise. (b) Intensity noise (spectral noise power, semi-logarithmic scale) as a function of the pump power for the same pillar under the same conditions as ina. The noise increases smoothly towards a peak just before the bistability threshold, then suddenly drops to form a gap where intensity squeezing is observed, with about the same value as ina. Here also the normalized spectral noise is obtained with three measurements (noise, shot noise and dark noise). In red is the curve obtained by increasing the pump power, in blue is the curve obtained by decreasing the pump power and the green line represents the shot noise (normalized to one). The thick black arrow points to whereawas recorded. (c) Bistability curve obtained by plotting the reflectance versus the pump power, for the same pillar under the same conditions as ina,b. The colour code is the same as inb. Above the thresholds the transmission is increased, hence a sharp reduction on the reflectance. Figure 3a,b shows the intensity noise measured with a balanced detection: a scan at fixed pump power in Fig. 3a and a scan of the noise versus pump power in Fig. 3b for a polariton–laser detuning Δ=0.19 meV that we have identified as optimal for squeezing. In Figs 3 and 4 the spectrum analyser was set to zero frequency span and centred at 7 MHz where the signal-to-noise ratio of the detection is maximum, with a sweep time ranging from 1 s to 20 s depending on the type of measurement. The resolution bandwidth (spectral bandwidth of the measurement) was 300 kHz with a 30 Hz video bandwidth (temporal integration over a 30 Hz bandwidth). For the noise dependence on the pump power ( Fig. 3b ), the motorized plate controlling the excitation power on the pillar is scanned at the same time as the spectrum analyser. We then compare the measured noise to the shot noise. The protocol involves recording the shot noise in difference mode, immediately switching to addition mode to record the intensity noise and then switching back to shot noise measurement (difference mode again) in order to check its stability. The dark noise was recorded after each measurement by recording the electronic noise when the laser beam is blocked. All the presented noise measurements are obtained by normalizing the noise traces by the shot noise after subtraction of the dark noise from both the noise and the shot noise. Figure 3: Intensity squeezing and bistability. ( a ) Squeezed intensity noise at fixed pump power near the lower turning point (linear scale), on a 6 μm pillar at cavity–exciton detuning of −5 meV and a polariton–laser detuning of 0.19 meV. The noise data were normalized with a measurement of the shot noise and a measurement of the dark noise, with S ( t ) = (noise( t ) −<dark( t )>)/(< shotnoise( t )>−<dark( t )>), <...> being the time average. The measured noise reduction is 20.3±1.5% (−1 dB) below the shot noise limit before corrections, 35.8±2.6% after. The dashed green line is the average noise and the red line is the shot noise. ( b ) Intensity noise (spectral noise power, semi-logarithmic scale) as a function of the pump power for the same pillar under the same conditions as in a . The noise increases smoothly towards a peak just before the bistability threshold, then suddenly drops to form a gap where intensity squeezing is observed, with about the same value as in a . Here also the normalized spectral noise is obtained with three measurements (noise, shot noise and dark noise). In red is the curve obtained by increasing the pump power, in blue is the curve obtained by decreasing the pump power and the green line represents the shot noise (normalized to one). The thick black arrow points to where a was recorded. ( c ) Bistability curve obtained by plotting the reflectance versus the pump power, for the same pillar under the same conditions as in a , b . The colour code is the same as in b . Above the thresholds the transmission is increased, hence a sharp reduction on the reflectance. Full size image A slight energy detuning between the pump laser and the ground state of the lower polariton branch gives rise to optical bistability [13] (see Fig. 3c ), characteristic in Kerr nonlinear media. According to theoretical predictions, the best squeezing rate is expected in the vicinity of the turning points of the bistability, as in other nonlinear systems [33] . We therefore chose to sweep the pump power in the vicinity of the bistable region (noise profile measurement, Fig. 3b ) to identify the best working points and we performed noise measurements with a fixed pump power corresponding to the maximum of intensity squeezing (steady-state measurement, Fig. 3a ). Squeezing was achieved in a reproducible way in repeated experiments on several different neighbouring pillars. According to previous calculations [34] the best squeezing is expected for a slightly negative cavity–exciton detuning (0> δ >−1 meV) in planar microcavities. Here the spatial confinement of pillars tends to enhance the polariton–polariton nonlinear interactions with respect to planar microcavities due to the increase in polariton density. We hence chose to work at larger negative cavity–exciton detuning ( δ ≈−5 meV) to have a larger photonic fraction, while preserving strong enough nonlinearities from the excitonic component. Experimental and theoretical results The strongest noise reduction at fixed pump power was obtained with the laser energy blue-detuned by about Δ=0.19 meV from the polariton lower energy level on a 6 μm pillar with a cavity–exciton detuning at δ ≈−5 meV. The measured intensity squeezing is 20.3±1.5%, as shown in Fig. 3a . After correction for detection efficiency (81%) and transmission losses ( T =70%), we infer a squeezing in the outgoing field of 35.8±2.6%. This result was established with a laser intensity lock reducing the low frequency (0–100 kHz) intensity variations to 0.2%. The use of the spatial filter was found not to be crucial, as the laser spot was well matched to the size of the six pillars. On the other hand, excessive spatial filtering led to a reduction of the squeezing, as expected from increasing losses. A coupled exciton–photon model with pump, losses and Kerr nonlinearity (described in Methods) predicts a squeezing value under these conditions of about 40%, in agreement with the experimental value. Effect of the pump–polariton detuning The values of pump power at which the optimal working points occur as well as the specific shape of the bistability curve depend on Δ. This parameter is also expected to influence the intensity noise profile and the squeezing value. The noise dependence on the pump power for the same pillar and parameter values as mentioned above is shown in Fig. 3b . Outside of the bistable region there is an excess noise due to thermal exciton reservoir populated by the pump laser. In the vicinity of the bistability thresholds, this noise undergoes amplification or deamplification due to the nonlinear effects. The intensity noise strongly increases below the bistability thresholds then decreases, as observed in other nonlinear systems [16] , [33] , [34] . At higher values of Δ, the pump power required to reach the bistability threshold increases and the noise profiles are drastically altered. Indeed a bistable behaviour appears above some critical value of Δ. For rather large Δ only the lower turning point (reached by decreasing the pump power) is able to produce intensity squeezing. If Δ is lower than the critical value, strong nonlinear modifications of the noise and reflectance can be observed despite the lack of bistable behaviour and the noise curves are the same when increasing or decreasing the pump power. These effects were studied in our experiment by repeating the noise measurements at different polariton–laser detunings and are discussed in the Supplementary Note 1 . Supplementary Figs 1 and 2 show, respectively, the reflectance and the noise plots obtained for Δ=0.10 meV while Supplementary Figs 3 and 4 show, respectively, the reflectance and the noise plots obtained for Δ=0.21 meV and Supplementary Figs 5 and 6 show the reflectance and the noise plots obtained for Δ=0.30 meV. The optimal detuning for squeezing that we present here corresponds to the onset of the bistability behaviour where the hysteresis cycle is very narrow ( Fig. 3b ). Homodyne detection To confirm these findings, we have measured the noise along all the field quadratures with the homodyne detection and checked that squeezing occurs only in the amplitude quadrature at the bistability turning points. As previously mentioned, for low Δ the output of the pillar is nearly Gaussian. In such conditions, we were able to achieve good mode matching between the local oscillator and the spatial mode emitted by the micropillar (about 90%) and implement an efficient homodyne detection. The path difference between the two beams, set to change linearly with time, determines the measured quadrature. The result is presented in Fig. 4 for a laser–polariton detuning of Δ=0.10 meV. Squeezing is observed at the minima of the curve showing the characteristic arches. Let us note that the anti-squeezed quadrature (phase quadrature) exhibits a large excess noise of the order of 12 dB due to thermal noise input. The fluctuations and irregularities of the noise arches are due to the fact that the interferometric homodyne set-up is more sensitive to mechanical instabilities. A comparison with the intensity measurements set-up allows checking that the squeezed quadrature indeed corresponds to the amplitude quadrature. The observed squeezing with this set-up was of about 16% (25% inferred after corrections). 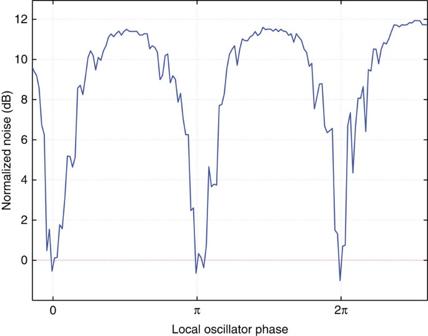Figure 4: Homodyne detection. Experimental measurement of squeezing with homodyne detection for a pump–polariton detuning of 0.10 meV on the same pillar as inFig. 3. The minima were verified to be in the amplitude quadrature. The squeezing obtained from the average between the values at 0,πand 2 π is 16% (−0.75 dB) before corrections and 25% after corrections. The reduced value of the squeezing here is mainly due to the non-optimal laser–polariton detuning. Figure 4: Homodyne detection. Experimental measurement of squeezing with homodyne detection for a pump–polariton detuning of 0.10 meV on the same pillar as in Fig. 3 . The minima were verified to be in the amplitude quadrature. The squeezing obtained from the average between the values at 0, π and 2 π is 16% (−0.75 dB) before corrections and 25% after corrections. The reduced value of the squeezing here is mainly due to the non-optimal laser–polariton detuning. Full size image In conclusion, we have reported an experimental demonstration of strong enhancement of squeezed light generation with confined polaritons in semiconductor micropillars. The best intensity squeezing was inferred to be 35.8±2.6% below the shot noise limit and was confirmed by measurements with a homodyne detection set-up. Several original optimizations allowed to reach these results. In particular, the special design of the pillars ensures a near-perfect mode matching between the pump and the polariton field; the discretization of the polariton energy modes allows for a strong reduction of the excess noise coming from phonon coupling. The reduced reflectivity of the upper Bragg mirror relative to that of the bottom mirror enhances the emission of light towards the top of the pillar, optimizing the light collection. Finally the relatively low-quality factor of the cavity increases the radiative to non-radiative losses ratio which, together with the choice of a working point with a high photonic fraction, results in a larger squeezing in the emitted light. These results demonstrate the improvement of intensity-squeezed light and light–matter fields brought by reduced dimensionality in semiconductor microstructures and open the way to the realization of ultra-low threshold integrated sources for the quantum information-processing technology. Theoretical model Owing to the lateral confinement of the micropillar, the polariton modes are well identified and we can selectively pump a polariton mode by tuning the spatial and spectral profile of the pumping light. For the theoretical analysis, we simply consider a single-cavity mode with frequency ω c and an exciton state with frequency ω x . The Hamiltonian of the coupled system (polariton) in the microcavity is: Here, and are the annihilation operators of a photon and an exciton, respectively, and Ω R is the coupling strength (vacuum Rabi splitting) between the cavity photon and the exciton. The last term represents a third-order nonlinearity for the excitons with strength g . The polaritons are subject to an effective Kerr effect through it. In addition, considering the photonic and excitonic reservoirs, the quantum Langevin equations for the cavity photons and the excitons are, respectively, derived as follows: Here, κ and γ are the dissipation rates of the cavity photon and exciton, respectively. and are the input operators from photonic and excitonic reservoirs, respectively, and we assume they have a zero average =0 (incoherent input). Instead, we explicitly consider an applied coherent pumping with amplitude F p and frequency ω p . Then, the input–output relation for the photon operators is expressed as: From the above Langevin equations, we first calculate the mean fields of the cavity photon and exciton induced by the coherent pump. Assuming and , the steady-state mean fields are as follows: Once the mean fields are determined, the reflectance is calculated via the input–output relation as follows: The intensity noise is calculated by the fluctuations around the mean field value. Defining the fluctuation operators as δ − α and δ − β , and linearizing the corresponding equations, the quantum Langevin equations are rewritten as follows: From these equations and the input–output relation, we can infer the fluctuations δ − α out of the output photons. The variance of the output is expressed as follows: Then, the normalized intensity noise is expressed as follows: The correlations of the output are calculated from the ones of input operators. Here, we assume that the correlation of the photonic input as (extracavity photon vacuum) while the excitonic reservoir has an incoherent population, namely = N th δ ( t − t ′) and =0. We also assume that there is no correlation between the photonic and excitonic inputs. N th represents the thermal noise and is chosen to be linear with the pump power ( N th = σ · W p (mW), with σ the proportionality constant and W p the pump power). Parameters In the calculations, we have used the following values: δ = ω c − ω x =−5 meV, Ω R =4 meV and κ =0.11 meV. The other parameters have been estimated by fitting experimental data for several values of Δ, the pump–polariton detuning and are shown in Table 1 . From the theoretical results of this simple model, we observe that the excitonic dissipation rate γ tends to increase with Δ. This can be explained by an increased population in the excitonic reservoir. Table 1 Parameters. Full size table This model is able to reproduce correctly the reflectance traces obtained in the experiment, and the intensity noise for pump intensities above the bistability threshold. Note that the prediction of the intensity noise for low pump intensities does not reproduce well the experimental data. This is probably due to the fact that our model does not take disorder effects into account. For very low densities, the disorder becomes the dominant effect, so we cannot capture the corresponding noise behaviour adequately. Supplementary Fig. 7 shows the comparison between the model and the experiment for the intensity noise at Δ=0.15 meV. The bistability curve of the reflectance and the corresponding intensity noise dependence on the pump power for a pump–polariton detuning of 0.26 meV are shown in Supplementary Fig. 8 and in Supplementary Fig. 9 , respectively. How to cite this article: Boulier, T. et al. Polariton-generated intensity squeezing in semiconductor micropillars. Nat. Commun. 5:3260 doi: 10.1038/ncomms4260 (2014).